Two-step synthesis of chiral fused tricyclic scaffolds from phenols via desymmetrization on nickel Tricyclic furan derivatives with multiple chiral centers are ubiquitous in natural products. Construction of such tricyclic scaffolds in a stereocontrolled, step-economic, and atom-economic manner is a key challenge. Here we show a nickel-catalyzed highly enantioselective synthesis of hydronaphtho[1,8- bc ]furans with five contiguous chiral centers via desymmetrization of alkynyl-cyclohexadienone by oxidative cyclization and following formal [4 + 2] cycloaddition processes. Alkynyl-cyclohexadienone was synthesized in one step from easily accessible phenols. This reaction represents excellent chemo-selectivity, regio-selectivity, diastereo-selectivity, and enantio-selectivity (single diastereomer, up to 99% ee). An extraordinary regioselectivity in the formal [4 + 2] cycloaddition step with enones revealed the diverse reactivity of the nickelacycle intermediate. Desymmetrization of alkynyl-cyclohexadienones via oxidative cyclization on nickel was supported by the isolation of a nickelacycle from a stoichiometric reaction. Enantioenriched tricyclic products contain various functional groups such as C=O and C=C. The synthetic utility of these products was demonstrated by derivatization of these functional groups. Hydronaphtho[1,8- bc ]furan rings with multiple chiral centers are a common structural motif in biologically active natural products (Fig. 1 a) [1] , [2] , [3] , [4] , – [5] . Such tricyclic structures are also found in key synthetic intermediates that are employed in a large number of sesquiterpenoids [6] , [7] , [8] , [9] . Owing to diverse biological activities and synthetic potentials associated with these fused tricyclic structures, a significant amount of attention has been paid to their enantioselective syntheses. Despite the existence of various stepwise stereoselective methods [1] , [2] , [3] , [4] , [5] , [6] , [7] , [8] , [9] , direct access to such tricyclic fused rings in a completely enantio-controlled, diastereo-controlled, step-economic, and atom-economic manner would be a remarkable development [10] , [11] , [12] , [13] . Recently, Alemán reported a straightforward method for the construction of tricyclic fused rings from a cyclohexadienone tethered alkenal by employing an organocatalyzed asymmetric desymmetrization strategy (Fig. 1b ) [14] . In this process, desymmetrization step involved the intramolecular [4 + 2] cycloaddition of chiral dienamine with a diastereotropic enone constructed tricyclic fused rings with three chiral centers. Fig. 1 Hydronaphtho[1,8- bc ]furans and their syntheses from phenols. a Representative examples of biologically active compounds. b Previous work employed desymmetrization by intramolecular [4+2] cycloaddition, catalyzed by organocatalyst. c Present work employed desymmetrization by oxidative cyclization and following intermolecular formal [4+2] cycloaddition process with nickel Full size image We envisaged the enantioselective desymmetrization [15] , [16] , [17] , [18] , [19] of alkynyl-cyclohexadienone via an intramolecular oxidative cyclization on nickel in the presence of a chiral ligand. Alkynyl-cyclohexadienone were synthesized in one step from easily accessible phenols. The oxidative cyclization of an enantiotropic enone with a tethered alkyne unit would form a tricyclic fused nickelacycle [20] , [21] , [22] , [23] , [24] with three chiral centers, which could react with another olefin to yield a tricyclic product with the concomitant generation of two more chiral centers. Nickel(0)-catalyzed trimerization of an alkyne with two enones has been reported by Montgomery et al. [25] , [26] , [27] , [28] and by us [29] , [30] . Here, we report a nickel(0)-catalyzed enantioselective synthesis of chiral hydronaphtho[1,8- bc ]furans with five contiguous chiral centers via desymmetrization of alkynyl-cyclohexadienone and following intermolecular formal [4 + 2] cycloaddition reaction processes. Reaction optimization Prior to developing the reaction in an asymmetric fashion, achiral ligands were examined using cyclohexadienone-yne ( 1a ) and 4-methoxychalcone ( 2a ) for the model transformation to hydronaphtho[1,8- bc ]furan 3aa (Fig. 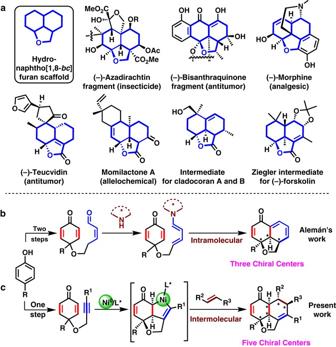Fig. 1 Hydronaphtho[1,8-bc]furans and their syntheses from phenols.aRepresentative examples of biologically active compounds.bPrevious work employed desymmetrization by intramolecular [4+2] cycloaddition, catalyzed by organocatalyst.cPresent work employed desymmetrization by oxidative cyclization and following intermolecular formal [4+2] cycloaddition process with nickel 2 , see also Supplementary Table 1 for detail). 1,3-Bis-(2,6-diisopropylphenyl)imidazol-2-ylidene (IPr) proved to be an optimal ligand to deliver rac - 3aa in 96% yield, whereas PCy 3 failed to give any product. A single diastereomer of 3aa was obtained out of sixteen possible isomers. Moreover, it is remarkable that an extraordinary regioselectivity was observed in the formal [4 + 2] cycloaddition step, fixing two carbonyls at the 1,4-positions in 3aa , whereas 1,5-dicarbonyl compounds were obtained in reports of nickel(0)-catalyzed cycloaddition reactions [20] , [21] , [22] , [23] , [24] , [25] , [26] , [27] , [28] , [29] , [30] . Considering the efficiency of N -heterocyclic carbene (NHC) in this transformation, chiral ( R , R )-NHCs, generated in situ by treating the corresponding imidazolinium salts with NaO t Bu, were investigated to afford enantioenriched 3aa (Fig. 2 ). It is worth mentioning that despite much exploration of the use of chiral NHCs, there has been less reports with nickel-catalyzed reactions [31] , [32] , [33] , [34] , [35] , [36] , [37] , [38] , [39] , [40] . N -(2-Biphenyl)- ( L*1 ) and N -(2-isopropylphenyl)- ( L*2 ) substituted NHCs [41] were ineffective to give 3aa . In a similar manner, N -(2,7-diisopropylnaphthyl)- ( L*4 ) [42] and N -(2,7-dicyclohexylnaphthyl) ( L*5 ) [34] -substituted NHCs also failed to yield any products. However, N -2,6-diethylphenyl-substituted NHC ( L*3) [43] successfully gave hydronaphtho[1,8- bc ]furan 3aa in 13% yield with high enantioselectivity (94% ee). NHCs L*6 [35] and L*7 [34] furnished 3aa in moderate chemical yields (36 and 48%, respectively) with excellent enantioselectivities (98 and 89% ee, respectively). Given the excellent enantioselectivity with L*6 , extensive effort was devoted to improving the yield. When the reaction was conducted at 60 °C using a lower concentration (0.02 M of 2a ), 3aa was obtained in 74% yield with 98% enantioselectivity (see Supplementary Table 1 for detail). Fig. 2 Evaluation of Ligands. ( R , R )- L*n ·HBF 4 , NaO t Bu, Ni(cod) 2 (0.01 mmol each), 1a (0.12 mmol), 2a (0.10 mmol), and toluene (1.0 ml) are employed. Isolated yields are given and enantioselectivity was determined by SFC equipped with a chiral stationary phase. a Yield and enantioselectivity was measured at 27% conversion in 3 days. b 5 ml toluene was employed and reaction was conducted at 60 °C. c 10 mol% IPr was used instead of chiral NHC salt and NaO t Bu. d 20 mol% PCy 3 was used instead of chiral NHC salt and NaO t Bu Full size image Substrate scope With the aforementioned optimal reaction conditions, we explored the scope of substrates (Fig. 3 ). A range of electron-rich and electron-deficient aryl-substituted enones 2 was examined with 1a . The reaction proceeded smoothly with 2b and 2c , giving 3ab and 3ac in 73 and 72% yields, respectively, with enantioselectivities of 98% each. Reaction with an enone containing 2-furyl group ( 2d ) was also examined with 1a to afford 3ad in 72% yield with 99% ee. In contrast, the reaction of 1a with 1-aryl-2-buten-1-ones ( 2e – 2i ) gave 3ae – 3ai in slightly lower yields (62–70%), albeit enantioselectivities remained excellent (94–97% ee). In these cases, about 5% of fully- intermolecular [2 + 2 + 2] cycloaddition products ( 3′ ) of an alkyne unit of dienone-yne ( 1a ) with two enones ( 2e – 2i ) were observed (See Supplementary Fig. 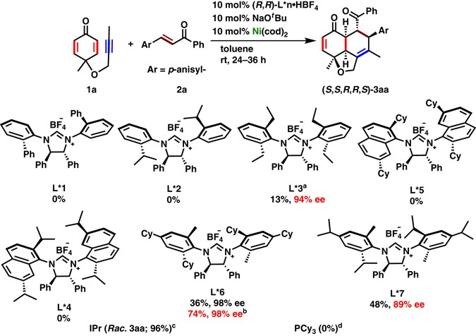Fig. 2 Evaluation of Ligands. (R,R)-L*n·HBF4, NaOtBu, Ni(cod)2(0.01 mmol each),1a(0.12 mmol),2a(0.10 mmol), and toluene (1.0 ml) are employed. Isolated yields are given and enantioselectivity was determined by SFC equipped with a chiral stationary phase.aYield and enantioselectivity was measured at 27% conversion in 3 days.b5 ml toluene was employed and reaction was conducted at 60 °C.c10 mol% IPr was used instead of chiral NHC salt and NaOtBu.d20 mol% PCy3was used instead of chiral NHC salt and NaOtBu 10 for 3ae′ ). When ethyl group at R 3 of an enone was introduced, a complex mixture was obtained. Next, alkynyl-cyclohexadienone substrates ( 1 ) were investigated by varying the substituents R 1 and R 2 . Ethyl as well as 2-methoxyethyl-substituted alkynyl-cyclohexadienone ( 1b and 1c ) gave 3bb , 3bj , 3ca , and 3ck with 2b , 2j , 2a , and 2k , respectively in good yields (60–73%) with excellent enantioselectivities (96–99%). Aryl and alkyl groups on alkynes were also examined. Phenyl-acetylene-substituted dienone 1d gave 3de in good yield with excellent enantioselectivity (70% yield and 99% ee). Electron-rich anisyl-group substrate 1e gave 3ec (71% yield and 98% ee) and 3ek (68% yield and 99% ee) with p -halogenated (F– and Cl–) chalcones 2c and 2k , respectively. No corresponding dehalogenated products were detected. An alkynyl-dienone 1f bearing an electron-deficient p -CO 2 EtC 6 H 4 – group gave 3fc with 2c in 60% yield with 98% ee, whereas 3ge was obtained in 71% yield with 96% ee from p -CF 3 -substituted 1g . An ethyl-group and a triethylsilyloxy-methyl-substituted alkynyl-cyclohexadienone ( 1h and 1i , respectively) gave corresponding tricyclic fused rings 3he , 3ic , and 3ik with 2e , 2c , and 2k , respectively, in good yields and enantioselectivities (69–77% yields, 95–98% ee). A N -tosyl analog of alkynyl-cyclohexadienone 1j failed to give the desired product 3jc with 2c under the present reaction conditions. This could have been due to coordination ability of tosyl group to nickel which inhibits the coordination of 2c [44] , [45] . The absolute configurations of all five chiral centers in 3 were assigned according to an analogy with 3ik , which was unambiguously determined by X-ray crystallographic analysis (Fig. 3 ). It also supports all the stereo selective and regioselective outcomes in 3 . Fig. 3 Substrate Scope. Reaction was examined at 0.1−0.4 mmol scale. Isolated yields are given and enantioselectivity was determined by SFC equipped with a chiral stationary phase. ORTEP diagram of 3ik is shown with thermal ellipsoid at 30% probability level. Hydrogen atoms are omitted for clarity except those bound to the chiral carbon centers. Flack parameter for 3ik = 0.017(7) Full size image Gram scale synthesis and transformations of product 3aa To demonstrate applicability, a half-gram-scale reaction of 1a (0.53 g, 3.0 mmol) was carried out with 2a (0.6 g, 2.5 mmol) to afford 3aa in 73% yield and 98% ee. These enantioenriched tricyclic products could be useful synthetic intermediates for further transformations (Fig. 4 ). The methylene group of a tetrahydrofuran ring was oxidized with PCC [46] to yield a butyrolactone scaffold ( 4 , 90% yield), that is present in natural products and also is a key synthetic intermediate in many sesquiterpenoids (Fig. 1a ) [6] , [7] , [8] , [9] . Epoxidation and Michael addition of an enone gave the corresponding functionalized products 5 and 6 as single diastereomers in 75 and 85% yields, respectively, whereas hydrogenation of an enonic C = C bond with H 2 /Pd(C) in ethyl acetate gave 7 in 89% yield. 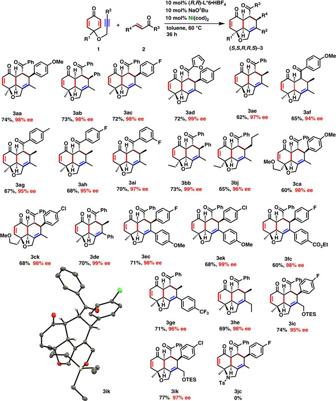Fig. 3 Substrate Scope. Reaction was examined at 0.1−0.4 mmol scale. Isolated yields are given and enantioselectivity was determined by SFC equipped with a chiral stationary phase. ORTEP diagram of3ikis shown with thermal ellipsoid at 30% probability level. Hydrogen atoms are omitted for clarity except those bound to the chiral carbon centers. Flack parameter for3ik= 0.017(7) The enantioselectivity remained consistent in all these transformations. Fig. 4 Synthetic Transformation of 3aa . Isolated yields are given and enantioselectivity was determined by SFC equipped with a chiral stationary phase Full size image Stoichiometric experiment In order to gain deeper insight into a possible reaction mechanism, stoichiometric experiments were conducted in C 6 D 6 . An attempts to isolate a chiral nickelacycle corresponds to 1g using an optimal NHC L*6 and Ni(cod) 2 was unsuccessful. 19 F NMR spectra showed seven peaks, revealed the existence of several intermediates, in which one of them might be much more reactive leads to desired product in the presence of an enone. However, an η 3 -oxaallyl nickelacycle ( 8 ) was isolated in 99% yield when a stoichiometric reaction of 1a was conducted with IPr and Ni(cod) 2 . The molecular structure of 8 was confirmed by X-ray crystallography (Fig. 5 ). The 1 H, 13 C, and 2D NMR analyses of 8 demonstrated that its structure in solution was consistent with that observed in crystal lattice. The reaction of 8 with 2e gave rac - 3ae in 95% isolated yield, which supported that desymmetrization by oxidative cyclization would play a key role in the present transformation. Fig. 5 Stoichiometric reaction with 1a . Isolated yield of 8 and rac - 3ae are given. The molecular structure of η 3 -cyclohexadienyl Ni-complex 8 is disordered and one of the disordered structure is depicted for simplicity with thermal ellipsoid at 30% probability level. i Pr groups and hydrogen atoms (except those bound to the chiral carbons) are omitted for clarity Full size image A plausible reaction mechanism is drawn on the basis of the results of the stoichiometric experiment and previous reports (Fig. 6 ) [20] , [21] , [22] , [23] , [24] , [25] , [26] , [27] , [28] , [29] , [30] , [33] , [34] , [35] , [36] , [37] , [38] , [39] , [40] , [41] , [42] . First, the intramolecular oxidative cyclization of 1 via the simultaneous coordination of an alkyne and an enantiotropic enone to the chiral Ni(0)/ L * species gives a desymmetrized nickelacycle A , which would be in equilibrium with its η 3 -oxaallylnickel structure A′ . Coordination of 2 to nickel center of A giving B , followed by insertion through a Ni–C sp 2 bond could form a thermodynamically favorable η 3 -oxaallylnickel structure either C or C′ . Then, a subsequent reductive elimination could afford a tricyclic fused structure 3 as a single diastereomer with the regeneration of nickel(0) species. Fig. 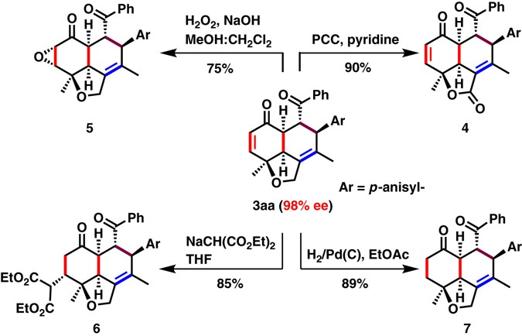Fig. 4 Synthetic Transformation of3aa. Isolated yields are given and enantioselectivity was determined by SFC equipped with a chiral stationary phase 6 A plausible reaction mechanism. Nickelacycle A is generated by enantioselective desymmetrization of 1 via oxidative cyclization. Subsequent insertion of an enone 2 to A gives a tricyclic product 3 Full size image In conclusion, a catalytic enantioselective method has been developed for the rapid construction of hydronaphtho[1,8- bc ]furans with five contiguous chiral centers via desymmetrization of alkynyl-cyclohexadienone and formal [4 + 2] cycloaddition reaction with nickel. The synthetic utility of tricyclic products was also demonstrated. Isolation of desymmetrized η 3 -oxaallyl nickelacycle and subsequent reactions in the stoichiometric experiment revealed that desymmetrization by oxidative cyclization is the key in this transformation. Furthermore, unusual regioselectivity in the insertion step of enone revealed the diverse reactivity of an η 3 -oxaallyl nickel-complex. The developed strategy involving two steps from the easily accessible phenols, demonstrates a practical and step economic protocol to access synthetically valuable fused tricyclic frameworks bearing five consecutive chiral carbon centers with excellent enantioselectivities. General procedure for tricyclic product 3 To a screw cap vial in a glove box was added L*6 ·HBF 4 (10 mol%) and NaO t Bu (10 mol%) and toluene (5 ml). The suspension was allowed to stir at room temperature for 10 min and then Ni(cod) 2 (10 mol%) was added. After further stirring for 10 min at room temperature was added a solution of alkynyl-cyclohexadienone ( 1 , 0.24 mmol) and enone ( 2 , 0.20 mmol) in toluene (5 ml). The reaction mixture was taken out of glove box and heated at 60 °C for 36 h with stirring. After cooling to room temperature, the mixture was filtered through celite and washed with Et 2 O. The filtrate was concentrated in vacuo and the residue was purified by silica gel flash chromatography (5–20% ethyl acetate in hexane) to afford the desired product 3 . Data availability The X-ray crystallographic coordinates for structures reported in this study have been deposited at the Cambridge Crystallographic Data Centre (CCDC) under deposition numbers CCDC 1523827 ( 3ik ) and 1523828 ( 8 ). These data can be obtained free of charge from The CCDC via www.ccdc.cam.ac.uk/data_request/cif . All other data supporting the findings of this study are available within the article and its Supplementary Information file or from the authors upon reasonable request. For NMR spectra of the compounds in this article, see Supplementary Figs. 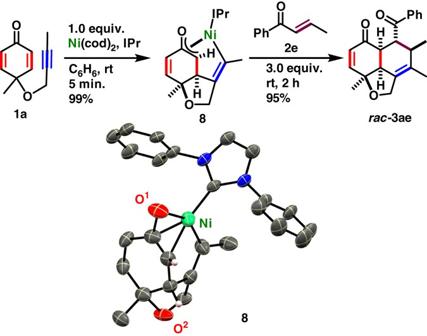Fig. 5 Stoichiometric reaction with1a. Isolated yield of8andrac-3aeare given. The molecular structure of η3-cyclohexadienyl Ni-complex8is disordered and one of the disordered structure is depicted for simplicity with thermal ellipsoid at 30% probability level.iPr groups and hydrogen atoms (except those bound to the chiral carbons) are omitted for clarity 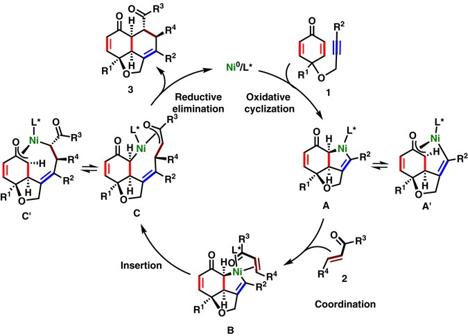Fig. 6 A plausible reaction mechanism. NickelacycleAis generated by enantioselective desymmetrization of1via oxidative cyclization. Subsequent insertion of an enone2toAgives a tricyclic product3 2 – 31 .